High-resolution nanotransfer printing applicable to diverse surfaces via interface-targeted adhesion switching Nanotransfer printing technology offers outstanding simplicity and throughput in the fabrication of transistors, metamaterials, epidermal sensors and other emerging devices. Nevertheless, the development of a large-area sub-50 nm nanotransfer printing process has been hindered by fundamental reliability issues in the replication of high-resolution templates and in the release of generated nanostructures. Here we present a solvent-assisted nanotransfer printing technique based on high-fidelity replication of sub-20 nm patterns using a dual-functional bilayer polymer thin film. For uniform and fast release of nanostructures on diverse receiver surfaces, interface-specific adhesion control is realized by employing a polydimethylsiloxane gel pad as a solvent-emitting transfer medium, providing unusual printing capability even on biological surfaces such as human skin and fruit peels. Based on this principle, we also demonstrate reliable printing of high-density metallic nanostructures for non-destructive and rapid surface-enhanced Raman spectroscopy analyses and for hydrogen detection sensors with excellent responsiveness. Ultra-high-resolution nanofabrication has become essential for the development of future devices in the deep-nanoscale regime, such as transistors [1] , [2] , sensors [3] , [4] , generators [5] , nonvolatile nanomemories [6] , nanowire photovoltatics [7] , metamaterials [8] , [9] and plasmonic devices [10] , [11] . The core elements in these devices with unprecedented performance are nanofabricated functional materials such as nanoparticles, nanowires and nanoribbons, which exhibit fundamentally different physical properties and functionalities from bulk materials [12] , [13] . For example, junction-free compact transistors can be realized using semiconducting nanowires with sub-20-nm dimensions [14] , and gas sensors for trace-amount detection can be fabricated using nanowire arrays with an exceptionally high surface-to-volume ratio [3] . The utilization of the quantum size effect from nanomaterials with sub-10 nm dimension can also facilitate the development of novel devices with unusual functionalities [12] , [13] , [15] . Furthermore, the high flexibility of nanomaterials makes them suitable for high-end flexible/stretchable electronics [3] , [16] , [17] . Among various emerging nanofabrication techniques, nanotransfer printing (nTP) has received considerable attention because it can readily generate highly functional nanostructures with two- and three-dimensional (3D) arrangements in a low-cost and high-throughput manner [18] , [19] , [20] . Most importantly, nTP holds potential as a practical method for the fabrication of flexible nanodevices because of its patterning capability on various substrates including flexible plastic substrates and non-planar surfaces [21] , [22] , where conventional patterning technologies are not easily applied. During the implementation of nTP, nanostructures are generated through vapour-phase or solution-phase deposition of functional materials on an elastomeric mold and subsequent transfer onto other substrates using a direct contact mechanism [18] , [19] , [20] . For this purpose, conventional nTP methods generally use surface-patterned elastomeric molds (for example, crosslinked polydimethylsiloxane (PDMS)) with low surface energy, which facilitates the release of nanostructures [18] , [20] . To date, there have been many reports on applications of nTP for practical device fabrications [23] . One example is 3D stacking of metallic and dielectric structures for the fabrication of metamaterials operating in the infrared range, a study reported by Rogers and co-workers [23] . Recently, the same group reported transfer printing of metal electrodes on human skin and demonstrated a prototype epidermal electronic system that can measure electrical signals from muscles [24] , [25] . Various nTP methods developed so far have, however, struggled with important remaining challenges. First, the ultimate resolution of nTP is determined by the resolution of the elastomeric replica stamp. Although considerable effort has been devoted to enhancing the resolution of nTP [26] , [27] , the resolution limit of the state-of-the-art nTP technology is still roughly 50 nm [28] . Further enhancement of resolution below 10 nm would make it possible to fabricate nano-devices with better performance by exploiting the quantum size effect and enhanced integration densities. We previously reported a means of circumventing these issues by transfer printing μm-wide block copolymer (BCP) thin film stripes containing ordered sub-10 nm microdomains [21] . However, this method requires the repetition of BCP self-assembly and additional pattern-transfer processes based on material deposition and dry etching for the fabrication of functional nanostructures. Second, the direct deposition of ‘ink materials’ on elastomeric stamps often fails in terms of reliable printing of nanostructures onto receiver substrates because of adhesive interactions between the mold and deposited materials. To circumvent these obstacles, additional treatments such as heat treatment [29] , surface oxidation [19] and the use of self-assembled monolayers [20] and liquid bridges [28] , [30] are generally required in previous studies, making the overall process more complicated and limiting the choice of receiver substrates. Third, elastomers of low surface energy also have low moduli, which can result in merging of surface topographic patterns of a replica stamp during transfer printing [31] . This inevitably lowers the fabrication yield and registration quality of transferred nanostructures. Here we introduce a sub-20 nm (down to 9 nm) transfer printing method based on the adoption of a disposable polymer thin film replica and interface-targeted injection of solvent molecules for dynamic adhesion control. This nano-to-macro-scale printing method can be used for the fabrication of diverse structures in a size range from sub-10 nm to micrometres. We show how the injection of plasticizing solvent molecules from a PDMS gel pad can controllably weaken the adhesion to allow reliable and on-demand release of ultrafine nanostructures. The orders-of-magnitude decrease in peel strength and interfacial fracture energy that enable the fast and high-yield transfer-printing mechanism can be explained by the solvent-assisted change of interfacial friction energy. This strategy of switchable adhesion control is effective for various types of functional materials and receiver substrates including plastic substrates and even human skin and nail surfaces. Based on this new nTP approach, we demonstrate a fast and non-destructive surface-enhanced Raman spectroscopy (SERS) analysis and the fabrication of hydrogen sensors on nonplanar substrates and flexible substrates as example applications to show the utility and feasibility of this method for device fabrication and other applications. Solvent-assisted transfer printing of sub-20 nm nanowires The procedure for solvent-injection-assisted nTP (S-nTP), which is composed of two sequential steps, is schematically illustrated in Fig. 1 . In step 1 (pattern replication and transfer-printing of nanowires on a flexible substrate), the surface patterns on a master substrate are replicated by coating a polymeric thin film, and peeling off the film using a polyimide (PI) adhesive film. This replication process circumvents the need of repeating high-resolution lithography (KrF photolithography and BCP self-assembly in this study) for the fabrication of a master mold. We employed directed self-assembly of polystyrene- b -polydimethylsiloxane (PS- b -PDMS) BCPs, which we previously reported [32] , [33] , for large-area preparation of a high-resolution master mold (see Methods). The original master templates were used many times without degradation because the replication process does not require the application of pressure or heat. It should also be noted that this thin-film-based replication process can significantly save the amount of required materials compared with the typical fabrication processes for bulk replicas. Nanostructures can then be formed by depositing functional materials on the thin film replica. The nanowires formed on flexible substrates obtained by the step 1 process can be directly used for flexible device fabrications as will be shown at the later part. 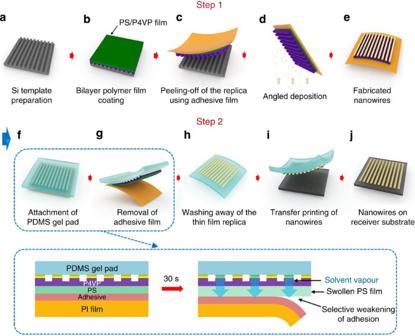Figure 1: Procedure for solvent-assisted nanotransfer printing. Step 1 (ultra-high-resolution replication and transfer printing onto a flexible substrate) is composed of (a) master mold fabrication by photolithography (μm ranges) or block copolymer self-assembly (8–20 nm), (b) replication using a bilayer (polystyrene (PS)/poly(4-vinyl pyridine) (P4VP)) polymer thin film, (c) peeling-off of the replica using a polyimide (PI) adhesive film, and (d,e) nanostructure formation on the replica via the angled deposition of functional materials. Step 2 (transfer printing to arbitrary substrates) entails (f) contact of solvent-swollen polydimethylsiloxane (PDMS) gel pad on the nanostructures to be transferred, (g) removal of adhesive film by weakening the PS/PI film adhesion through the incorporation of solvent molecules from the gel pad, (h) elimination of polymer replica (PS/P4VP) by solvent-washing and (i–j) transfer-printing of the functional nanostructures on various substrates by making contacts. Figure 1: Procedure for solvent-assisted nanotransfer printing. Step 1 (ultra-high-resolution replication and transfer printing onto a flexible substrate) is composed of ( a ) master mold fabrication by photolithography (μm ranges) or block copolymer self-assembly (8–20 nm), ( b ) replication using a bilayer (polystyrene (PS)/poly(4-vinyl pyridine) (P4VP)) polymer thin film, ( c ) peeling-off of the replica using a polyimide (PI) adhesive film, and ( d , e ) nanostructure formation on the replica via the angled deposition of functional materials. Step 2 (transfer printing to arbitrary substrates) entails ( f ) contact of solvent-swollen polydimethylsiloxane (PDMS) gel pad on the nanostructures to be transferred, ( g ) removal of adhesive film by weakening the PS/PI film adhesion through the incorporation of solvent molecules from the gel pad, ( h ) elimination of polymer replica (PS/P4VP) by solvent-washing and ( i – j ) transfer-printing of the functional nanostructures on various substrates by making contacts. Full size image Additional step 2 process (transfer printing on arbitrary substrates) can be continued when the nanostructures are needed to be transferred to other substrates. A PDMS gel pad prepared by immersing dry PDMS in a solvent is brought into contact with the nanostructures on the replica. Then, the solvent-saturated PDMS pad emits solvent molecules from its surface, which can effectively and selectively plasticize the top layer of the bilayer polymer replica and weaken the adhesion of the adhesive film, eventually transferring the nanostructures and the polymer replica to the surface of PDMS gel pad by removal of the adhesive film. After selectively washing away the organic replica using appropriate solvents, nanostructures on the PDMS pad (universal transfer medium) can be transfer printed onto various substrates via a short (~1 s) contact and release process. The master substrates were prepared by patterning the surface of a silicon wafer through photolithography and/or BCP lithography followed by plasma etching [32] , [34] . In particular, we employed BCP nanolithography for the fabrication of 8–20 nm scale templates [33] , [35] ; the detailed fabrication process is presented in the Methods section. It should be noted that BCP self-assembly can also generate other types of geometries such as nanoscale dots, holes and rings [35] , [36] , [37] . As will be shown, S-nTP is effective regardless of the dimensions of the master mold patterns from sub-10 nm range to μm dimensions. The surface of the master mold was treated with a low-surface-tension ( γ =20 mN m −1 ) PDMS brush to enable facile release of the polymer replica film from the master mold. For preparation of the disposable polymer replica, polystyrene (PS)/poly(4-vinyl pyridine) (P4VP) bilayer thin films were spin-coated sequentially on the functionalized master mold (See the Methods section for more details). The two polymeric thin films have respective functions in the pattern replication and the release of the replica from an adhesive film. First, P4VP provides ultra-high (sub-10 nm) replication resolution, thus effectively replicating surface patterns of master substrates down to a sub-10 nm scale. Second, PS was employed because it can easily be detached from the adhesive film by penetration of toluene molecules into the PS/adhesive film interface. The proper selection of detachment polymer layer (PS) and corresponding good solvent (toluene) successfully realized this strategy of interface-targetted adhesion switching. The extremly limited solubility of P4VP in toluene, contrary to the case of PS [38] , can securely maintain the alignment of the functional nanostructures. 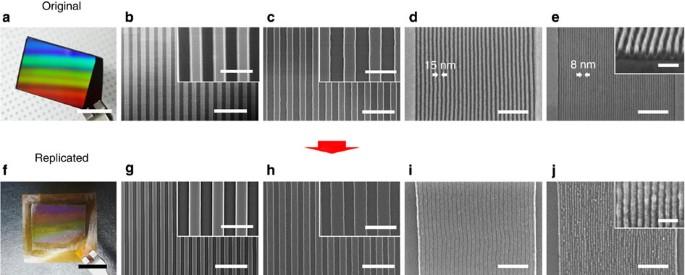Figure 2: Preparation of polymer thin film replica. (a) Photograph of original master substrate with periodic surface patterns. (b–e) SEM images of surface grating patterns of master substrates with line widths of (b) 2 μm, (c) 200 nm, (d) 15 nm and (e) 8 nm. (f) Optical image of the polymer replica prepared via step 1. (g–j) Corresponding SEM images of grating patterns of the replica with widths of (g) 2 μm, (h) 200 nm, (i) 20 nm and (j) 9 nm. Scale bar, 1 cm (a,f), 15 μm (b,g), 5 μm (insets inb,g), 1 μm (c,h), 500 nm (insets inc,h), 200 nm (d,e,i,j) and 50 nm (insets ine,j). Figure 2 shows optical and scanning electron microscope (SEM) images of the surface patterns of the master substrates in a wide size range from 8 nm to 2 μm and their corresponding polymer replica patterns peeled off the master mold substrates. In particular, Fig. 2i,j show that the bilayer polymer thin film successfully replicated high-resolution BCP nanopatterns with widths of 15 nm ( Fig. 2d ) and 8 nm ( Fig. 2e ), respectively. In this study, we largely focused on the fabrication of sub-20 nm-scale functional nanostructures using BCP nanotemplates and their replicas. Figure 2: Preparation of polymer thin film replica. ( a ) Photograph of original master substrate with periodic surface patterns. ( b – e ) SEM images of surface grating patterns of master substrates with line widths of ( b ) 2 μm, ( c ) 200 nm, ( d ) 15 nm and ( e ) 8 nm. ( f ) Optical image of the polymer replica prepared via step 1. ( g – j ) Corresponding SEM images of grating patterns of the replica with widths of ( g ) 2 μm, ( h ) 200 nm, ( i ) 20 nm and ( j ) 9 nm. Scale bar, 1 cm ( a , f ), 15 μm ( b , g ), 5 μm (insets in b , g ), 1 μm ( c , h ), 500 nm (insets in c , h ), 200 nm ( d , e , i , j ) and 50 nm (insets in e , j ). Full size image We confirmed that various metallic nanostructures can be formed through the direct deposition of materials onto the disposable polymer replica. In this step, we employed the glancing-angle deposition method, where the plane of the polymer replica substrate is not perpendicular to the deposition direction of the materials [39] , [40] , enabling the formation of discrete nanostructures on the replicas. The deposition angle from the substrate surface normal was modulated and optimized between 60° and 80°, depending on the pattern size and the template depth. By utilizing the shadowing effect during the oblique-angle deposition, discrete nanostructures were successfully prepared on the polymer replica without material residues in the recessed regions of the patterns. 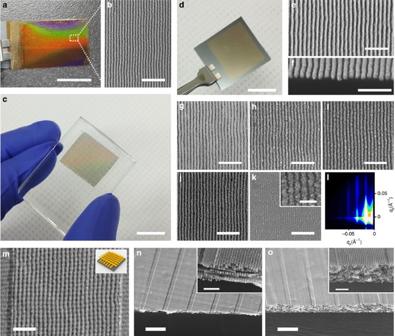Figure 3: Transfer-printed nanostructures via S-nTP. (a) Optical image showing the Au nanowires on replica/PI film prepared via angled deposition of the material. (b) Magnified SEM image of Au nanowires on the replica substrate. (c) Photograph of transferred Au nanowires onto PDMS pad. (d) An optical image showing Au nanowires transfer printed onto a Si wafer. (e) Top-down and (f) cross-section SEM images of the printed Au nanowires. (g–j) 20-nm-wide (g) Al, (h) Cu, (i) Ag and (j) Co-nanowires printed on a Si wafer. (k) 9-nm-wide Cr nanowires. (l) Grazing-incidence small-angle X-ray scattering (GISAXS) pattern of the printed Al nanowires. Three-dimensional superstructures can also be formed via multiple S-nTP. After the first printing of sub-20 nm nanowire arrays, the second printing was conducted by rotating the substrate by 90°, which resulted in crossed-wire structures. (m) Crossed-wire structure composed of two layers of 20-nm-wide gold nanowires. Multiple printing of nanowires resulted in more complicated three-dimensional structures. (n) Seven layers of crossed gold nanowires with a perpendicular arrangement between adjacent layers. (o) 20 layers of gold nanowires with a parallel arrangement. Scale bar, 1 cm (a,c,d), 1 μm (n,o) and 200 nm (b,e–k,m, insets inn,o). Figure 3a,b presents a gold-deposited polymer thin film replica on PI adhesive film and a magnified SEM image confirming the formation of 20-nm-wide gold nanowire arrays on the replica. Figure 3: Transfer-printed nanostructures via S-nTP. ( a ) Optical image showing the Au nanowires on replica/PI film prepared via angled deposition of the material. ( b ) Magnified SEM image of Au nanowires on the replica substrate. ( c ) Photograph of transferred Au nanowires onto PDMS pad. ( d ) An optical image showing Au nanowires transfer printed onto a Si wafer. ( e ) Top-down and ( f ) cross-section SEM images of the printed Au nanowires. ( g – j ) 20-nm-wide ( g ) Al, ( h ) Cu, ( i ) Ag and ( j ) Co-nanowires printed on a Si wafer. ( k ) 9-nm-wide Cr nanowires. ( l ) Grazing-incidence small-angle X-ray scattering (GISAXS) pattern of the printed Al nanowires. Three-dimensional superstructures can also be formed via multiple S-nTP. After the first printing of sub-20 nm nanowire arrays, the second printing was conducted by rotating the substrate by 90°, which resulted in crossed-wire structures. ( m ) Crossed-wire structure composed of two layers of 20-nm-wide gold nanowires. Multiple printing of nanowires resulted in more complicated three-dimensional structures. ( n ) Seven layers of crossed gold nanowires with a perpendicular arrangement between adjacent layers. ( o ) 20 layers of gold nanowires with a parallel arrangement. Scale bar, 1 cm ( a , c , d ), 1 μm ( n , o ) and 200 nm ( b , e – k , m , insets in n , o ). Full size image For secure transfer of the nanostructures to a PDMS substrate, which can serve as a universal transfer medium to any surface, we used a solvent-swollen PDMS substrate prepared by dipping a PDMS pad into a toluene (solubility parameter, δ =18.3 MPa 1/2 ) bath [38] for 6 h for full saturation ( Supplementary Fig. 1 ). When fully swollen in the toluene bath, the PDMS gel pad preserved its flatness and mechanical stability. In a previous work, we confirmed the preservation of shape, flatness and mechanical robustness of a swollen PDMS gel pad with a diameter of up to 300 mm (ref. 34 ). This solvent-immersion process can also prevent contamination of transfer-printed nanostructures because of uncrosslinked oligomers through their dissolution [41] . The solvent-swollen PDMS pad could be used for more than 1 h, which is much longer than the S-nTP-processing time (step 2 shown in Fig. 1 ) of less than 1–2 min without any noticeable deformation or change of curvature. The use of the PDMS gel pad provides dual functionality in terms of adhesion control. Immediately after attachment of the PDMS pad on the multilayer of metallic nanostructure/P4VP/PS/adhesive film, the solvent molecules spontaneously migrate from the PDMS gel to the targeted PS film ( δ =18.5 MPa 1/2 ) [41] and plasticize the PS film because of the high solubility of PS in toluene. The first role of the PDMS gel pad is significant weakening of the adhesion between the adhesive film and the PS layer. As a result of the weakened adhesion, the adhesive film can easily and cleanly be detached from the polymer replica without causing any damage to the P4VP replica or the functional nanostructures. The photograph in Fig. 3c shows PS/P4VP/nanostructures transferred onto a PDMS gel pad. The transferred PS/P4VP layer was dissolved away by dipping the PDMS into the solvent bath (toluene and isopropyl alcohol). During the replica removal process, delamination of the transferred nanostructures was not observed. Gentle washing of the polymer layers guaranteed 100% preservation of the nanostructures. The achievement of this simple and reliable solvent-assisted transfer process is important because this technique allows the facile release of polymer replicas from the original master templates using conventional adhesive films and also because reliable and fast removal of the adhesive film is possible. Moreover, this transfer mechanism based on solvent-assisted adhesion switching is clearly differentiated from the release of structures by the removal of a sacrificial layer, which is used for membrane fabrications, for example [42] . First, in contrast to the previous method, our approach does not permanently remove any components. This is substantiated by the observation that the weakened adhesive force is recovered by drying the solvent from the stacked structures (specifically from the adhesive and PS). This mechanism does not leave any residue, and thus the quality of transferred nanostructures is significantly improved. Second, Although the complete dissolution of a sacrificial layer requires at least centimetre-scale macroscopic diffusion of the solvent in the lateral direction and consequently long treatment time for complete removal of the layer, our approach is markedly faster because of shorter diffusion length (only tens of nm) along the surface-normal direction in the stack. By contacting the PDMS pad with various receiver substrates, the aligned metallic nanostructures were reliably transfer-printed without losing the degree of alignment or the mutual registration between them. The second role of the PDMS gel pad is to enable facile release of the nanostructures from its surface. Application of mild pressure (less than 20 kPa) ensured conformal contact between the PDMS pad and the receiver substrate, and the nanostructures were transferred onto the substrate almost instantly as soon as contact was made. As shown in Fig. 3d–f , we successfully printed 20-nm-wide gold nanowires on a silicon wafer. The width of the nanowires was dependent on the thickness of the films deposited by evaporation. By depositing various other materials on the replicated template, we could also fabricate and transfer-print perfectly aligned nanowires such as Cu, Al, Ag, Co and Cr ( Fig. 3g–k ). Because the polymer replica fabrication guarantees resolution below 10 nm, as shown above, S-nTP also worked in the sub-10 nm regime. We fabricated 9-nm-wide Cr nanowires using an 8-nm-wide BCP template and reliably transfer-printed the nanowires onto a Si wafer, as shown in Fig. 3k . We additionally evaluated and confirmed large-area uniformity of the printed nanowires through grazing-incidence small-angle X-ray scattering (GISAXS) measurement and a SEM image analysis. In addition to the SEM analysis results for several different locations ( Supplementary Fig. 2 ), the consistently well-resolved peaks in the GISAXS patterns shown in Fig. 3l and Supplementary Figs 3 and 4 also support the excellent uniformity and fidelity of S-nTP over a macroscopic area (2 × 1.5 cm 2 ). The original alignment of the printed nanowires was maintained and confirmed after the entire transfer-printing procedure including the removal process of the polymer replica and the transfer-printing process, and no buckling or wrinkling was observed in the printed nanowire structures from SEM characterizations. Importantly, excellent mechanical stability of the printed nanowires was confirmed from maintenance of the original arrangement after repeated peel tests using adhesive tape, as shown in Supplementary Fig. 5 . Mechanism of solvent-assisted adhesion control An S-nTP process with unprecedented high resolution and reliability was established through solvent-assisted control of adhesion between an adhesive film and a polymer replica, as schematically shown in Fig. 4a . As mentioned above, we observed that, for a dry state without the supply of a solvent, the adhesion between the adhesive film and the PS layer was stronger than that between nanostructures and a dry PDMS pad. However, the use of a PDMS gel pad emitting toluene resulted in abrupt switching of adhesive forces, that is, the adhesion of the adhesive interface became weaker than that of any other interfaces in the stacking structure. 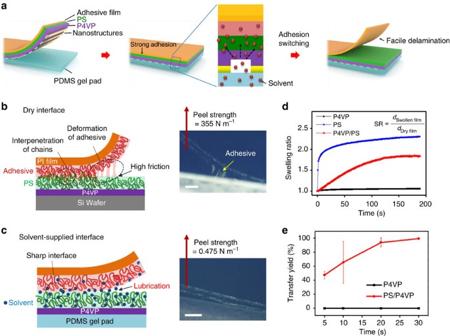Figure 4: The mechanism of solvent-assisted adhesion control. (a) Procedure of solvent-assisted adhesion control. The out-diffused solvent molecules enable facile delamination of the adhesive film from the polymer replicas. (b,c) Schematic illustrations describing adhesion mechanisms for (b) dry and (c) solvent-supplied interface between the adhesive film and PS layer. Although the cross-section photograph inbshows significant stretching of the adhesive because of strong adhesion, the corresponding image incdemonstrates clear-cut interfaces at a much lower peel strength with the assistance of solvent molecules. (d)In-situmeasured swelling ratio (SR=thickness of swollen film/thickness of dry film) of polymer films. TheSRof P4VP under saturated toluene vapour was approximately 1.05, whereas theSRof PS covered by P4VP under the same conditions was about 1.82, indicating significant swelling of PS by toluene molecules supplied through the thin (60 nm) P4VP layer. (e) Transfer yield of the nanostructures from the adhesive film to the PDMS gel pad depending on the supply time of toluene. The error bars indicate one standard deviation. Scale bar, 100 μm (optical images inb,c). Figure 4: The mechanism of solvent-assisted adhesion control. ( a ) Procedure of solvent-assisted adhesion control. The out-diffused solvent molecules enable facile delamination of the adhesive film from the polymer replicas. ( b , c ) Schematic illustrations describing adhesion mechanisms for ( b ) dry and ( c ) solvent-supplied interface between the adhesive film and PS layer. Although the cross-section photograph in b shows significant stretching of the adhesive because of strong adhesion, the corresponding image in c demonstrates clear-cut interfaces at a much lower peel strength with the assistance of solvent molecules. ( d ) In-situ measured swelling ratio ( SR =thickness of swollen film/thickness of dry film) of polymer films. The SR of P4VP under saturated toluene vapour was approximately 1.05, whereas the SR of PS covered by P4VP under the same conditions was about 1.82, indicating significant swelling of PS by toluene molecules supplied through the thin (60 nm) P4VP layer. ( e ) Transfer yield of the nanostructures from the adhesive film to the PDMS gel pad depending on the supply time of toluene. The error bars indicate one standard deviation. Scale bar, 100 μm (optical images in b , c ). Full size image In the case of peeling off an adhesive film from a substance, a crack first should be formed at the edge of the film and then should propagate until the entire film is separated from the substance. Such delamination occurs at the interface when the mechanically applied energy (fracture energy, G ) per unit increase of crack area is sufficiently large [43] , [44] . The fracture energy can be calculated by measuring the force applied during the peeling process. When peel strength ( P , peel force per unit width) is applied to the adhesive film ( Supplementary Fig. 6 ), a crack propagates with a uniform velocity, and the corresponding fracture energy ( G ) can be given as where E , h and θ are the elastic modulus, thickness of the PI backing film, and peel angle, respectively [44] , [45] . We measured P required to separate the adhesive and polymer film, and using equation(1), we calculated the fracture energy ( G adhesive-PS ) at the interface between the adhesive and PS for cases with and without a solvent supply. For measurement of dry-state G adhesive-PS , P4VP and PS films were sequentially spin-casted on a Si wafer, and a PI adhesive film was attached on the PS film, as schematically shown in Fig. 4b . In this case, a Si wafer was used as a substrate instead of dry PDMS because the adhesive force at the interface between P4VP and the Si wafer was stronger than that between the adhesive and PS, whereas that between P4VP and dry PDMS was weaker than the adhesive force of other interfaces. Thus, in the stacked structure shown in Fig. 4b , delamination occurs at the interface between the adhesive and PS, as intended, enabling measurement of dry-state G adhesive-PS . For measurement of P and G adhesive-PS under a solvent supply, the PDMS gel pad was brought into contact with the nanostructures/bilayer replica/adhesive film structure. The measured P adhesive-PS values were 355 and 0.475 N m −1 for the dry and wet interfaces, respectively, showing almost a three orders of magnitude decrease of peel strength by the use of the solvent-emitting PDMS pad. The corresponding dry-state G adhesive-PS was calculated to be 102 J m −2 , whereas G adhesive-PS dramatically decreased to a value of 0.136 J m −2 by the attachment of the PDMS gel pad. One factor affecting the G of a delaminated interface is the thermodynamic work of adhesion ( W a ), which can be defined as where γ adhesive , γ PS and γ adhesive-PS are surface energy terms of the adhesive, PS and the interface energy between them, respectively. However, the measured fracture energy at the dry state was more than three orders of magnitude higher than W a (<2 γ PS =80 mJ m −2 ). This huge difference is consistent with previous studies that reported a negligibly small contribution of W a in the fracture energy during the peeling of an adhesive from a surface [44] , [46] . Instead, a critical role of interfacial friction in the delamination of an adhesive from a substrate and its dominance in the fracture energy over W a have been reported in previous studies [44] , [47] . For initiation of the slip process and detachment of the adhesive, shear force applied on the interface should be higher than the maximum static frictional force, which is sufficiently high for viscoelastic adhesives to be deformed plastically by applied stress [45] , [47] , [48] . The frictional energy ( G f ) mentioned above can be expressed as where k =the kinetic friction coefficient, v =the slip velocity, and x =the distance from the crack tip, respectively [44] . In a dry state, the friction coefficient ( k ) at the adhesive and PS is high due to strong van der Waals interactions resulting from interpenetration of polymer chains [46] , [49] , [50] , [51] . Slippage of the adhesive layer thus would not occur before the application of sufficiently high P . Such high peel force also causes significant deformation of the adhesive, as shown in the photograph in Fig. 4b , which was obtained from the edge of the crack tip region while detaching the adhesive film. In contrast, in the case of solvent-assisted delamination, the adhesive film easily slips on the PS surface even with a small peel force. Note also that stretching or deformation of the adhesive was not observed, as is clearly visible in the optical image shown in Fig. 4c . The dramatic decrease in G adhesive-PS in the presence of the solvent can be understood by the marked decrease of k . When the solvent molecules are supplied, they can permeate through the P4VP film and selectively swell the PS film and adhesive ( Fig. 4c ). The solvent molecules present between the films cause hydrodynamic lubrication, and as a result the resistance to friction at the interface may be dramatically reduced. Extremely reduced friction between polymers swollen under a good solvent, the so called ‘super lubrication’ phenomenon, was reported in recent studies [52] , [53] . In the presence of a good solvent, the interpenetration between extended chains is highly suppressed because of a significant entropic penalty, and thus interfacial friction can be reduced by a factor of ~10 3 (refs 52 , 53 ). The assurance of significant swelling of two polymers where delamination occurs is thus the key condition for interface-specific control of adhesion for transfer printing. The remaining question here is whether toluene molecules from the PDMS gel pad can be supplied through P4VP with a low solubility in toluene. Using in-situ reflectometry measurement, we experimentally confirmed that the solvent molecules can permeate the P4VP replica and can swell the underlying PS film. As shown in Fig. 4d , the saturated swelling ratio ( SR , the solvent-swollen thickness divided by its dry thickness) under saturated toluene vapour for PS covered by P4VP was measured to be 1.82. This result substantiates that toluene molecules can migrate through the thin P4VP layer and arrive at the PS film, which is consistent with the phenomenon that molecules can diffuse through free volumes in polymers even in the case of low solubility [54] . The SR of the P4VP single-layer film under saturated toluene vapour was measured to be approximately 1.05, indicating 5% swelling of P4VP by saturated toluene vapour. Although this value is much lower than that of PS or PS/P4VP under the same environment, it still clearly indicates the permeation of toluene in P4VP. Moreover, the extremely small thickness (60 nm) of P4VP may allow easy passage of toluene across the P4VP layer. The transfer yield of the nanostructures from the adhesive film to the PDMS gel pad was highly dependent on the supply time of toluene vapour ( Fig. 4e ). We found that 30 s of solvent supply was sufficient for complete transfer of the nanostructures/polymer replica to the PDMS pad. However, without a supply of solvent vapour, they could not be transferred at all because the weaker adhesion between the nanostructures and dry PDMS prevented delamination of the adhesive from PS. The role of the solvent was also essential for the reliable transfer of nanostructures from the PDMS gel pad to arbitrary substrates after the removal of polymer thin film replicas. We calculated the fracture energy values for dry and gel-state PDMS on a stainless steel surface (an example of a metallic surface) by measuring P (peel strength). As shown in Table 1 , although the dry PDMS pad required a P of 6.94 N m −1 ( G =2.00 J m −2 ) for delamination, P for the PDMS gel pad was measured to be only 1.16 N m −1 ( G =0.332 J m −2 ). The significantly reduced adhesion between the nanostructures and the PDMS pad thus contributed to extremely facile and reliable transfer printing of ultrafine nanostructures onto various surfaces with a transfer yield of nearly 100%, even for a short contact duration time (1 s or shorter). As a comparison, when transfer-printing was performed after all of the solvent was removed from the samples, dry PDMS failed to enable transfer-printing of the ultrafine nanostructures, as shown in Supplementary Fig. 7 . These results validate the critical contributions of solvent molecules for interface-specific reduction of adhesion force and fracture energy and the achievement of reliable transfer-printing capability. Table 1 Measured peel strength ( P ) and calculated fracture energy ( G ) under dry and solvent-supplied conditions. Full size table S-nTP of metal nanowires onto diverse surfaces and SERS analyses One notable advantage of our S-nTP method is that it allows transfer-printing on almost arbitrary substrates because solvent molecules present on the wet PDMS facilitate the release of nanostructures from the pad to various receiver surfaces. S-nTP does not require any equipment or additional treatments, such as heat treatment, surface oxidation or use of self-assembled monolayers or liquid bridges, which previously were reported to be necessary in conventional nTP approaches for the transfer of nanostructures from a dry PDMS mold [23] , [24] , [28] , [35] . Our simple but universal approach—the use of a solvent-swollen PDMS gel pad instead of the conventional dry PDMS pad—can remove the aforementioned obstacles and allow the achievement of versatile, ultra-high-resolution sub-10 nm nTP. In addition to transfer onto flat substrates, as demonstrated in Fig. 3 , we also successfully transfer-printed gold nanowires onto the non-planar inner surface of a vial glass ( Fig. 5a,b ), ultra-thin flexible film ( Fig. 5h ), surface-patterned topographic substrate ( Fig. 5i ) and shrinkage film ( Fig. 5j ). More strikingly, S-nTP can be used for the generation of uniform and aligned nanostructures on highly complex biological substances including human fingernail ( Fig. 5c,d ), human skin (wrist, Fig. 5e,f ) and the surface of a fruit (apple, Fig. 5g ) without any substrate surface treatment. These results suggest that this new transfer-printing approach can contribute to the development of in vivo sensors that can detect and analyse biological signals and biomarkers. 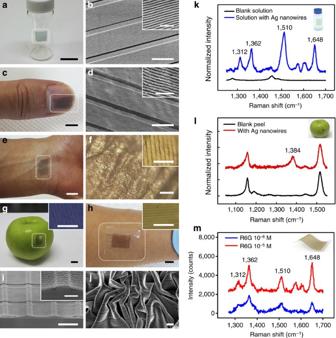Figure 5: S-nTP of metallic nanowires onto unusual surfaces. (a,b) Nonplanar glass vial, (c,d) human finger nail, (e,f) wrist skin, (g) surface of an apple, (h) flexible substrate attached on skin, (i) surface-patterned Si substrate and (j) shrinkage film. Scale bar, 1 cm (a,c,e,g,h), 100 μm (f), 5 μm (insets inf,g,h), 1 μm (b,d,i,j), and 200 nm (insets inb,d,i). (k) Raman signal spectra obtained from a vial glass containing 10−5M Rhodamine 6G (R6G) solution. The designated Raman signal peaks correspond to those of R6G. The printing of Ag nanowires on the inside surface of the vial significantly enhanced the signal intensity. (l) Raman signal obtained from the surface of an apple coated with Thiram (tetramethylthiuram disulfide) with an areal density of 1 μg cm−2. Raman signal peak at 1384, cm−1corresponds to that of Thiram. Although the characteristic peak of Thiram was not observed for the reference sample (Thiram-coated apple), Ag nanowire printing on the same sample enabled the detection of the peak. (m) Raman signal spectra obtained from a Ag-nanowire-printed PET film coated with 10−5–10−6M R6G solution. Figure 5: S-nTP of metallic nanowires onto unusual surfaces. ( a , b ) Nonplanar glass vial, ( c , d ) human finger nail, ( e , f ) wrist skin, ( g ) surface of an apple, ( h ) flexible substrate attached on skin, ( i ) surface-patterned Si substrate and ( j ) shrinkage film. Scale bar, 1 cm ( a , c , e , g , h ), 100 μm ( f ), 5 μm (insets in f , g , h ), 1 μm ( b , d , i , j ), and 200 nm (insets in b , d , i ). ( k ) Raman signal spectra obtained from a vial glass containing 10 −5 M Rhodamine 6G (R6G) solution. The designated Raman signal peaks correspond to those of R6G. The printing of Ag nanowires on the inside surface of the vial significantly enhanced the signal intensity. ( l ) Raman signal obtained from the surface of an apple coated with Thiram (tetramethylthiuram disulfide) with an areal density of 1 μg cm −2 . Raman signal peak at 1384, cm −1 corresponds to that of Thiram. Although the characteristic peak of Thiram was not observed for the reference sample (Thiram-coated apple), Ag nanowire printing on the same sample enabled the detection of the peak. ( m ) Raman signal spectra obtained from a Ag-nanowire-printed PET film coated with 10 −5 –10 −6 M R6G solution. Full size image We transfer-printed Ag nanowires onto a Si substrate and evaluated their SERS analysis performance by comparing the obtained SERS spectrum with that from a commercially available SERS substrate. The SERS substrate based on the transfer-printed Ag nanowires showed clearly resolved Raman peaks of rhodamine 6G (R6G) molecules even at a low concentration of 10 −9 M ( Supplementary Fig. 8 ), which is comparable with the best reported detection level [55] , [56] , [57] , [58] . It should be noted that the signal intensity obtained from the commercial SERS substrate at the same concentration was negligibly small. Moreover, the signals were highly uniform over a large area (~1 cm 2 ) with a standard deviation of 5–9%, as shown in Supplementary Fig. 9 . As an example of a near-term application, we demonstrate that Ag nanowires printed on the inner surface of a vial glass can enhance SERS signals, enabling direct and convenient detection of molecules dispersed in a solution at an extremely low concentration. The graph in Fig. 5k shows clearly resolved SERS peaks corresponding to Rhodamine 6G molecules dispersed in an ethanol solution with a concentration of 10 −5 M. As another example, transfer printing of Ag nanowires onto the surface of a fruit enables direct and rapid detection of pesticide residues on the surface using a SERS analysis, as shown in Fig. 5l . The detection of Thiram (tetramethylthiuram disulfide, a widely used pesticide/fungicide that can cause physical disorders of the human body by chronic or acute exposure) molecules was observed only when Ag nanowires were present on the apple surface. It should be also be emphasized that the areal density (1 μg cm −2 ) of the detected pesticide molecules on the apple peel in this work is even lower than the maximally permissible pesticide residue level for fruits (22~31 μg cm −2 ) [59] . (EU Pesticides database. http://ec.europa.eu/sanco_pesticides/public/?event=homepage , 05 September 2014.). The utilization of S-nTP can significantly enhance the analysis throughput of SERS by decreasing the analysis preparation time (for the attachment of plasmonic nanostructures on analytes) to 1 s. Although, for similar applications, the coating of colloidal nanoparticles can be considered, the complete drying of solvent would take at least tens of seconds and it would not be simple to reproducibly distribute plasmonic nanoparticles with a constant areal density. S-nTP also allowed printing of functional nanostructures onto ultra-thin and highly flexible plastic substrates. We demonstrated flexible SERS film based on Ag nanowires upon 10-μm-thick PET film, which could be wrapped around even human arms, as shown in Fig. 5h . Such flexible SERS film showed fairly high Raman signal enhancement, and SERS signals corresponding to R6G molecules from the solutions with concentration as low as 10 −6 M could be obtained ( Fig. 5m ) [60] . Our S-nTP technique also allows multiple, sequential printing for the fabrication of 3D nanostructures. Layer-by-layer printing of highly aligned nanostructures will open further opportunities in nanofabrication, for example, the realization of 3D multilayered superstructures. As a demonstration, we fabricated high-density (625 per μm 2 ) crossed-wire structures through sequential printing of aligned gold nanowires. After the first printing of 20-nm-wide nanowire arrays, a second printing step was conducted by rotating the substrate by 90°, which resulted in crossed-wire structures, as shown in Fig. 3m . Multiple printing of nanowires resulted in more complicated 3D structures. Figure 3n, o shows seven-layer-stacked crossed gold nanowires with a perpendicular arrangement between adjacent layers and 20-layer-stacked gold nanowires with a parallel alignment, respectively. Such multilayered superstructures can exhibit new functionalities not observed in conventional two-dimensional structures or thin films. For example, crossed magnetic nanowires can be endowed with stepwise magnetization behaviour because of different magnetization behaviour between the under and upper layers [61] , [62] . Such multilayered superstructures composed of sub-20 nm scale components may also have importance in the development of metamaterials operating in the ultraviolet–visible regime [63] , [64] . Demonstration of a flexible and printable hydrogen sensor We next demonstrate the fabrication of a flexible and printable sensor device using S-nTP. 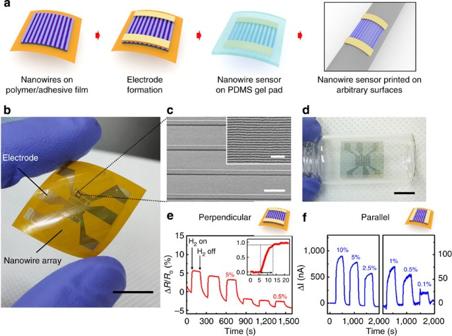Figure 6: Demonstration of flexible and printable hydrogen sensor. (a) Fabrication procedure for a two-terminal hydrogen sensor based on aligned Pd nanowires prepared by S-nTP. (b) A photograph of the fabricated flexible hydrogen sensor on a plastic substrate. (c) Magnified SEM image showing Pd nanowires between electrodes. (d) An optical image of a printed hydrogen sensor on a curved surface of a glass vial. (e–f) Performance of the hydrogen sensor device upon periodic supply of diluted H2gas with different concentrations. The alignment directions of Pd nanowires were (e) perpendicular to and (f) parallel with the electrodes, respectively. The inset ineshows the variation of the signal at 0.5% H2and indicates a response time (Rt) of 8 s. Scale bar, 1 cm (b,d), 1 μm (c) and 200 nm (inset inc). Figure 6a illustrates the fabrication procedure for an ultrafine palladium (Pd) nanowire sensor for hydrogen detection. First, a 20-nm-wide Pd nanowire array on a polymer replica on adhesive film was prepared through replication of a high-resolution BCP template and angled deposition of Pd. Electrode pads connecting the Pd nanowires were then formed by depositing Au in the presence of a shadow mask. The photograph in Fig. 6b shows the flexible nanowire sensor on a PI substrate. The high-magnification SEM images ( Fig. 6c ) obtained from the sensing region of the device show that the Pd nanowire array between the electrodes is uniformly formed with exceptionally good ordering. Figure 6: Demonstration of flexible and printable hydrogen sensor. ( a ) Fabrication procedure for a two-terminal hydrogen sensor based on aligned Pd nanowires prepared by S-nTP. ( b ) A photograph of the fabricated flexible hydrogen sensor on a plastic substrate. ( c ) Magnified SEM image showing Pd nanowires between electrodes. ( d ) An optical image of a printed hydrogen sensor on a curved surface of a glass vial. ( e – f ) Performance of the hydrogen sensor device upon periodic supply of diluted H 2 gas with different concentrations. The alignment directions of Pd nanowires were ( e ) perpendicular to and ( f ) parallel with the electrodes, respectively. The inset in e shows the variation of the signal at 0.5% H 2 and indicates a response time ( R t ) of 8 s. Scale bar, 1 cm ( b , d ), 1 μm ( c ) and 200 nm (inset in c ). Full size image For measurement of the hydrogen-sensing performance of the nanowire sensor, we monitored the resistance change ratio (Δ R / R o ) or the current change (Δ I ) of the device with flowing N 2 /H 2 mixing gas. Interestingly, two different hydrogen-sensing principles based on Δ R / R o and Δ I measurements can be exploited by a sensor based on aligned Pd nanowires. First, when the electrode pads were initially connected at the two ends of the Pd nanowires, the resistance increased as the hydrogen concentration in the mixing gas increased because of the higher resistivity of Pd hydride (PdH x ) compared with pure Pd [65] . In order to prevent the formation of β-phase and unfavourable large volume expansion [66] , [67] , the measurement was conducted at 60 °C. For this sensing principle, the measured Δ R / R o ( R o : initial resistance, Δ R : change of R from R o ) values were positive, as shown in Fig. 6e . The device was able to successfully detect H 2 gas at a concentration as low as 0.5%. Alternatively, when the Pd nanowires are aligned parallel with the border of the electrodes, most of the nanowires are not in contact with the electrodes, resulting in a very high R o . However, the volume expansion of the discrete Pd nanowires upon the uptake of hydrogen causes mutual contact and leads to the formation of electrically conducting paths between the electrodes [68] , and as a result positive Δ I values were obtained, as shown in Fig. 6f . Exceptionally narrow spacing (sub-20 nm) between Pd nanowires allowed a fast response of the device even under diluted (0.1%) hydrogen gas. The response time ( R t ) of a sensor is defined as the time required to reach 90% of the saturated value at the plateau. The measured R t was 8 s for the perpendicular device at 0.5% H 2 , as shown in the inset of Fig. 6e . Also, R t for the parallel device at 0.1% H 2 was measured to be 8 s. These response times are comparable with those reported in previous studies [69] . It also should be noted that the sensor device on the PI adhesive film is transferrable to other unconventional surfaces. For example, using the process depicted in Fig. 1 (step 2) employing a PDMS gel pad, we could successfully transfer print a Pd nanowire sensor even on the curved surface of a vial glass, as shown in Fig. 6d . These results strongly support our assertion that S-nTP is a simple, convenient and high-yield option to form devices on non-trivial surfaces. In summary, we have developed and presented a practical nano-transfer printing approach (S-nTP) that is effective in the sub-20 nm regime. Reliable replication of ultra-small (down to 8 nm) BCP nanostructures was realized via spin-casting of appropriate polymer thin films and subsequently peeling off the thin films using conventional adhesive film. We also showed that the spontaneous injection of a solvent from a PDMS gel pad into the interfaces between the polymer replica and PI film enabled facile switching of adhesion and on-demand release of functional nanostructures on diverse, unconventional substrates. This led to successful transfer-printing of ultrafine gold nanostructures even on human skin/nail and fruit peels. We also demonstrated the fabrication and operation of a hydrogen sensor based on transfer-printed Pd nanowires with controlled alignment directions with respect to electrodes. Three-dimensional superstructures such as multilayers of crossed and parallel nanowires and various hierarchical structures were also successfully fabricated through sequential transfer-printing. We expect that by further modulating the geometry of the original patterns and depositing various functional materials, diverse flexible and printable nano-devices can also be realized. This new nTP technology with sufficiently high resolution and outstanding versatility can be exploited for high-throughput fabrication of future devices with novel functionalities and high integration density and with greatly improved performance based on non-conventional platforms. Fabrication of μm-scale master mold The Si trench master mold with widths of 200 nm and 2 μm were fabricated using KrF photolithography followed by reactive ion etching. A positive photoresist (PR, Dongjin Semichem Co. Ltd.) with a thickness of 400 nm was spin-coated on 200 mm Si wafers. The PR film was then exposed using a KrF scanner (Nikon, NSR-S203B), followed by developing using a developer solution (tetramethylammonium hydroxide, Dongjin Semichem Co. Ltd.). The PR patterns were used as an etch mask to pattern the Si surface by reactive ion etching (gas: CF 4 , working pressure: 7 mTorr, plasma power: 250 W). Fabrication of sub-20 nm master mold SD16 (MW=16 kg mol −1 ) and SD45 (MW=45.5 kg mol −1 ) PS- b -PDMS BCPs, which form 8-nm-wide and 15-nm-wide lines, respectively, were purchased from Polymer Source Inc. and used without purification. SD16 BCP was dissolved in a mixed solvent of toluene, heptane and PGMEA (1:1:1 by volume), yielding a 0.8-wt% polymer solution. Surface-patterned Si substrates with a width of 1 μm, a depth of 40 nm, and a period of 1.25 μm were used as guiding templates. The substrate was treated with a PDMS brush (5 kg mol −1 , Polymer Source Inc.) at 150 °C using a vacuum oven. A solution of SD16 was spin-cast onto the template and was thermally annealed at 200 °C for 30 min using a vacuum oven. Similarly, SD45 was dissolved in a mixed solvent of toluene, heptane and PGMEA (1:1:1 by volume), yielding a 1.0-wt% polymer solution, which was spin-cast onto the template and annealed for 6 h in the chamber at room temperature using toluene vapour. In order to remove the top-segregated PDMS layer and organic block (PS), the samples were etched by CF 4 plasma (etching time=20 s, gas flow rate=30 s.c.c.m., working pressure=15 mTorr, and plasma source power=50 W) followed by O 2 plasma (etching time=30 s, gas flow rate=30 s.c.c.m., working pressure=15 mTorr and plasma source power=60 W). Replica fabrication from templates Before the replication, the surface of the master mold was treated with a PDMS brush (Polymer Source Inc.). P4VP (MW=60 kg mol −1 ) and PS (MW=35 kg mol −1 ) were purchased from Sigma Aldrich Inc., and they were dissolved in isopropyl alcohol (IPA) and toluene, respectively, to yield 2 wt% solutions. P4VP and PS films were sequentially spin-casted on the master mold at 4,000 RPM. A polyimide adhesive film (3M Inc.) was then attached on the surface of the bilayer polymer replica. By retracting the adhesive film from the mold, the replica with the inverted image of the templates’ surface topography was detached from the mold. Formation of functional nanostructures Various metallic nanostructures were formed through the glancing-angle deposition of materials onto the polymer replica using an e-beam evaporator. The deposition angle from the substrate surface normal was modulated and optimized between 60° and 80°, depending on the pattern size and the template depth. Preparation of PDMS gel pad Prepolymers and curing agent (Sylgard 184, Dow Corning Co. Ltd.) were mixed with a weight ratio of 10:1, and the resultant air bubbles in the mixture were eliminated by degassing under vacuum. The mixture was then poured onto a silicon wafer, and baked at 140 °C for 30 min using a convection oven. The prepared PDMS samples with a thickness of 15 mm were immersed in a bath of toluene for the preparation of gel pads. The fully swollen PDMS pads were removed from the solvent bath, and the solvent drops on the pads were immediately eliminated by gently blowing under nitrogen gas for 10 s. Transfer of nanostructures to PDMS pad The solvent-swollen PDMS pad was brought into contract with the nanostructure/P4VP/PS/PI adhesive film. After 30 s, the PI adhesive film was removed from the PDMS pad and the polymer film and the fabricated nanostructures were transferred to the surface of the pad. The polymer replica was dissolved by sequentially dipping it into the solvent baths (toluene and isopropyl alcohol, respectively). Printing of nanostructures onto receiver substrates The PDMS pad supporting the nanowires was brought into contact with various receiver substrates, and mild pressure (<20 kPa) was applied uniformly on the back side of the pad. After several seconds, the pad was retracted for transfer-printing. SERS measurement of R6G solution R6G was purchased from Sigma Aldrich. Inc. and was dissolved in ethanol to prepare a solution of 10 −5 M. Ag nanowires were printed on the inner surface of a vial glass, followed by filling the vial with an ethanol solution of R6G. The Raman scattering signal was collected for 30 s using a dispersive Raman microscope (ARAMIS Inc.) equipped with a 514-nm Ar-ion laser. Detection of pesticide residues on fruit peels Tetramethylthiuram disulfide was purchased from Sigma Aldrich. Inc. and was dissolved in tetrahydrofuran. A volume of 50 μl of the solution was dropped onto the surface of an apple, which was subsequently dried to yield an areal density of thiram of 1 μg cm −2 . Ag nanowires were then directly transfer printed onto the apple surface, followed by SERS measurement for 30 s. SEM characterization For the observation and analysis of the samples, a field emission SEM (Hitachi S-4800) with an acceleration voltage of 15 kV and a working distance of 5 mm was used. In-situ measurement of SR of polymer films The thickness variation of the polymer films (P4VP and PS) under a solvent-saturated PDMS gel pad was measured using a reflectometer (F20-UV, Filmetrics Inc.) with a measurement wavelength range of 350–1,100 nm. How to cite this article: Jeong, J. W. et al. High-resolution nanotransfer printing applicable to diverse surfaces via interface-targeted adhesion switching. Nat. Commun. 5:5387 doi: 10.1038/ncomms6387 (2014).